AtALMT9 is a malate-activated vacuolar chloride channel required for stomatal opening inArabidopsis Water deficit strongly affects crop productivity. Plants control water loss and CO 2 uptake by regulating the aperture of the stomatal pores within the leaf epidermis. Stomata aperture is regulated by the two guard cells forming the pore and changing their size in response to ion uptake and release. While our knowledge about potassium and chloride fluxes across the plasma membrane of guard cells is advanced, little is known about fluxes across the vacuolar membrane. Here we present the molecular identification of the long-sought-after vacuolar chloride channel. AtALMT9 is a chloride channel activated by physiological concentrations of cytosolic malate. Single-channel measurements demonstrate that this activation is due to a malate-dependent increase in the channel open probability. Arabidopsis thaliana atalmt9 knockout mutants exhibited impaired stomatal opening and wilt more slowly than the wild type. Our findings show that AtALMT9 is a vacuolar chloride channel having a major role in controlling stomata aperture. Water availability is critical for crop production. It has been predicted that climate change will bring drought to increasing areas of our arable lands and strategies to produce more drought tolerant plants are critical to future crop improvement ( http://ressources.ciheam.org/om/pdf/a80/00800414.pdf ). Stomata have a central role in regulating CO 2 uptake required for photosynthesis and water consumption in response to changing environmental conditions [1] , [2] , [3] , [4] , [5] . The aperture of the stomatal pore is regulated by changes in the osmotic potentials of the guard cells. These changes are mainly achieved by ion transport across cellular membranes [3] , [4] , [6] , [7] , [8] . Cells contain organic as well as inorganic anions, both of which are of primary importance for stomatal opening and closure [1] , [4] , [6] , [8] , [9] . Potassium uptake from the apoplast and its accumulation in the vacuole are crucial during stomatal opening [1] , [4] , [7] . This process can only be achieved by a concomitant accumulation of anions, which allow balancing positive charges. The chemical nature of the anions involved in stomatal movements depends on the plant species and the growing conditions [10] , however it is generally accepted that chloride, malate and nitrate are the major actors [2] , [4] , [11] . Surprisingly, despite the importance of anion transport, until recently the molecular identity of these transporters remained elusive. In the last decade, the CLC [12] , [13] , SLAC [8] , [9] , [14] and ALMT [15] , [16] , [17] , [18] , [19] , [20] protein families have been found to be involved in the transport of anions, shedding light on the nature of anion fluxes across plant vacuolar and/or plasma membranes [11] . Despite the fundamental role of the vacuole in accumulating solutes during stomatal movement, none of the mutant plants of the so far identified anion transporters and channels displayed a visible phenotype. AtCLCc represents the only exception by exhibiting slightly impaired stomatal movement in epidermal strips [13] . Surprisingly, no genuine vacuolar chloride ion channel has been identified at the molecular level to date and only few reports of chloride channel activity on a functional level exist [21] , [22] . Among the anion transporter/channel families identified so far, aluminium-activated malate transporters (ALMTs) form a unique family of passive transport systems that are exclusive to plants [15] , [16] , [17] , [18] , [19] . Plasma membrane-located ALMTs are involved in dicarboxylic acid excretion required for aluminium tolerance and in the efflux of inorganic and organic anions during stomatal closure generating the well-described R-type current [17] . The first characterized ALMT in the tonoplast was AtALMT9, which has been shown to mediate malate and fumarate currents directed into the vacuole of mesophyll cells of Arabidopsis thaliana [18] . Subsequently, a second member, AtALMT6, was shown to mediate Ca 2+ - and pH-dependent malate currents into guard cell vacuoles [19] . Despite the fact that AtALMT6 is expressed nearly exclusively in guard cells, no obvious phenotype was observed. This may be due to the complex regulation of this ALMT. In general, ALMTs present a complex selectivity with a preference for dicarboxylic acids. However, the maize ALMT protein ZmALMT1 [23] has been shown to transport exclusively inorganic anions across the plasma membrane of root cells. In contrast, none of the vacuolar ALMTs was unambiguously demonstrated to mediate inorganic anion fluxes [18] , [19] . The scarce information concerning vacuolar chloride channels prevents the understanding of the physiology of this anion in plants. This is especially true if we consider the impact of the transport of chloride during salt stress tolerance and in mediating stomatal movements [6] , [8] , [9] , [11] , [24] . Here we show that the major role of AtALMT9 is to act as a malate-induced chloride channel. Chloride currents mediated by AtALMT9 are modulated by cytosolic malate concentrations in the physiological range. In planta AtALMT9 is required for proper regulation of stomata opening. Knockout plants for AtALMT9 exhibit a reduced stomata aperture and slower opening kinetics leading to plants with a reduced transpiration level, thus resulting in more drought tolerance than the corresponding wild types. AtALMT9 is permeable to chloride To re-evaluate whether AtALMT9 is able to transport chloride, we applied an electrophysiological approach using vacuoles isolated from protoplasts of Nicotiana benthamiana transiently overexpressing AtALMT9. To identify the transformed vacuoles, we expressed AtALMT9 fused to GFP at the C-terminus. Whole-vacuole measurements on these tobacco plants displayed a high malate current density [18] . To distinguish anion currents from background cation currents, we designed measuring solutions with the major cation being BisTrisPropane (BTP). BTP is largely impermeable, thus minimizing the cation current contribution in our measurement [12] , [19] . AtALMT9-mediated currents in the excised out-side-out configuration using symmetrical malate concentrations (100 mM Malate cyt /100 mM Malate vac ) displayed time-dependent relaxations similar to those previously observed for the vacuolar AtALMT9 [18] and AtALMT6 [19] . Differently from AtALMT6, AtALMT9 is not regulated by cytosolic Ca 2+ ( Supplementary Fig. S1 ). The mean amplitude of the AtALMT9-mediated currents under these ionic conditions was −1.8±0.6 nA at –120 mV ( Fig. 1a ), the currents displayed an inward rectification ( Fig. 1b ) and a reversal potential of 0±1 mV. Subsequently, we investigated whether chloride is permeable through AtALMT9. Therefore, we performed experiments in which the cytosolic buffer was exchanged with 100 mM Cl − ( Fig. 1a ). After this exchange, we could observe a current that was 13.5±3% of the current measured in presence of malate. The current was inward rectifying and detectable at membrane potentials more negative than −60 mV. Moreover, we found that the chloride currents were characterized by a higher noise compared with those observed for malate ( Fig. 1a ). These data indicate that AtALMT9 is permeable to chloride and mediates its transport from the cytosol to the vacuolar lumen. To ensure that the chloride currents were not due to a background activity, we compared patches from N. benthamiana vacuoles expressing AtALMT9-GFP with patches from N. benthamiana vacuoles expressing the empty vector using symmetrical chloride buffers (100 mM Cl cyt − /100 mM Cl vac − ). The patches expressing AtALMT9-GFP displayed time-dependent relaxation and a total current amplitude of −866±150 pA, while empty-vector-transformed patches exhibited no time-dependent relaxation and a total current amplitude of −70±32 pA ( Fig. 1c ). Taken together, these data show that AtALMT9 is not only a malate channel but is also able to transport chloride. Interestingly, chloride fluxes through AtALMT9 are hallmarked by a high level of fluctuations ( Fig. 1a ). 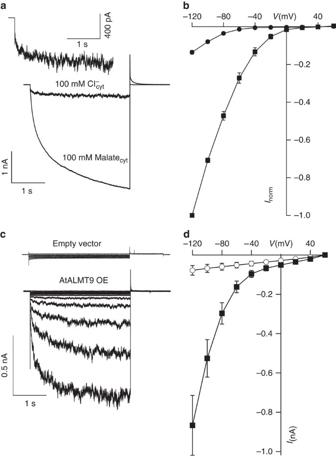Figure 1: AtALMT9 mediates chloride transport across the vacuolar membrane. (a) Excised cytosolic-side-out patches fromN. benthamianadisplay time-dependent currents in symmetrical malate conditions (100 mM malatecyt/100 mM malatevac; currents evoked in response 3-s pulse at −120 mV followed by a tail pulse at +60 mV, holding potential +60 mV). When cytosolic malate is exchanged with chloride the inward currents decrease and present an increased noise level (upper, curve enlargement of the chloride current). (b) NormalizedI–Vcurves of vacuolar patches from AtALMT9 overexpressingN. benthamianaplants in presence of 100 mM malate (squares;n=8) or 100 mM chloride (circles;n=8) at the cytosolic side (Supplementary Fig. S10; non-normalizedI–Vcurves). (c,d) In presence of symmetrical chloride conditions (100 mM Clcyt−/100 mM Clvac−; −120 mV), only cytosolic-side-out patches from vacuoles isolated from AtALMT9 overexpressingN. benthamianaplants present time-dependent relaxation (c). Total inward currents were ~10 times higher in cytosolic-side-out patches from AtALMT9 overexpressing vacuoles than in patches from empty-vector-transformed vacuoles. (c) Representative currents measured in vacuolar patches from empty-vector-transformed (upper trace) and from AtALMT9 overexpressing plants (lower trace), currents evoked in response 3-s pulse from +60 mV to −120 mV in −20 mV steps, followed by a tail pulse at +60 mV, holding potential −60 mV. (d)I–Vcurves measured in vacuolar patches from empty-vector-transformed (open circles; n=6) and from AtALMT9 overexpressingN. benthamianaplants (square; n=16). Error bars represents s.e.m. Figure 1: AtALMT9 mediates chloride transport across the vacuolar membrane. ( a ) Excised cytosolic-side-out patches from N. benthamiana display time-dependent currents in symmetrical malate conditions (100 mM malate cyt /100 mM malate vac ; currents evoked in response 3-s pulse at −120 mV followed by a tail pulse at +60 mV, holding potential +60 mV). When cytosolic malate is exchanged with chloride the inward currents decrease and present an increased noise level (upper, curve enlargement of the chloride current). ( b ) Normalized I – V curves of vacuolar patches from AtALMT9 overexpressing N. benthamiana plants in presence of 100 mM malate (squares; n =8) or 100 mM chloride (circles; n =8) at the cytosolic side ( Supplementary Fig. S10 ; non-normalized I – V curves). ( c , d ) In presence of symmetrical chloride conditions (100 mM Cl cyt − /100 mM Cl vac − ; −120 mV), only cytosolic-side-out patches from vacuoles isolated from AtALMT9 overexpressing N. benthamiana plants present time-dependent relaxation ( c ). Total inward currents were ~10 times higher in cytosolic-side-out patches from AtALMT9 overexpressing vacuoles than in patches from empty-vector-transformed vacuoles. ( c ) Representative currents measured in vacuolar patches from empty-vector-transformed (upper trace) and from AtALMT9 overexpressing plants (lower trace), currents evoked in response 3-s pulse from +60 mV to −120 mV in −20 mV steps, followed by a tail pulse at +60 mV, holding potential −60 mV. ( d ) I – V curves measured in vacuolar patches from empty-vector-transformed (open circles ; n =6) and from AtALMT9 overexpressing N. benthamiana plants (square ; n =16). Error bars represents s.e.m. Full size image Cytosolic malate is an activator of AtALMT9 Analysing the time course during the exchange in more detail, we observed that during the exchange of the cytosolic buffer from 100 mM malate to 100 mM Cl − , the fluctuation level of the current raised before it reached a stationary level ( Fig. 2a ). This behaviour attracted our attention. Indeed, the presence of this marked fluctuation indicated that the current is likely to be mainly mediated by Cl − ions, although a certain concentration of malate might be still present at the cytosolic side. After an increase in the noise level, the current continued to decline until it reached a steady state when only chloride was present ( Fig. 2a ). Therefore, we hypothesized that cytosolic malate may not only be a substrate for AtALMT9 but exhibits an additional function. Consequently, we tested whether cytosolic malate was able to modulate AtALMT9-mediated chloride currents. When we exchanged the 100 mM Cl cyt − buffer with a 100 mM Cl cyt − plus 1 mM malate cyt membrane patches from N. bethamiana overexpressing AtALMT9, we observed a stunning increase of the inward currents of 3.7±0.3 times ( Fig. 2b ). In contrast, in patches from empty-vector-transformed vacuoles, no current increase was observed after the application of 1 mM malate cyt ( Supplementary Fig. S2 ). These results proved that cytosolic malate is able to activate AtALMT9-mediated chloride currents. The currents measured in presence of 1 mM malate exhibited high fluctuations like those in the absence of malate ( Fig. 2b ). Moreover, the I / V characteristics showed that the activation triggered by the presence of 1 mM cytosolic malate shifted the threshold of activation from −60 mV to −40 mV ( Fig. 2c ). This shift of the activation threshold makes AtALMT9-mediated chloride transport physiologically even more relevant, as it occurs at vacuolar membrane potentials in a physiological range [4] . The kinetic analysis of the malate activation demonstrated that malate is an allosteric activator of AtALMT9 ( Fig. 2d ). The activation was well described by a Hill equation with coefficient n H =2.5 and an EC 50 =300 μM at −120 mV ( Fig. 2d ). These data provide two important disclosures: (i) they suggest that AtALMT9 is likely to be a multimeric complex with a number of subunits higher or equal than the Hill coefficient n H , and (ii) they show that the EC 50 of the activation by malate is within the physiological range of cytosolic malate concentration, which was reported to be between 400 and 800 μM (refs 25 , 26 , 27 ). This strongly suggests that AtALMT9 acts as a malate-activated vacuolar chloride channel in vivo , as the K m for malate transport is 27 mM ( Supplementary Fig. S3 ), a value far away from the cytosolic malate concentrations. To test the activation effect of other dicarboxylates, we tested whether fumarate, oxaloacetate and glutamate were able to activate AtALMT9-mediated chloride currents ( Fig. 2e ). While fumarate and oxaloacetic acid stimulated the chloride fluxes, though at different extents (5.7±0.4 and 2.0±0.2 times, respectively), the amino acid glutamate was ineffective in stimulating chloride transport ( Fig. 2e ). It indicates that the interaction and the effect of dicarboxylic acids on AtALMT9 activity depend on the structural characteristics of the agonist. This observation is similar to that made for ligand activated channels where different agonists exhibit different degrees of activation [28] . Taken together, our data clearly demonstrate that AtALMT9 is allosterically activated by cytosolic dicarboxylates, especially malate and fumarate. However, it does not answer the question whether the site of interaction is at the cytosolic or at the vacuolar side. Indeed, as effective agonists such as malate and fumarate permeate through AtALMT9, it would be possible that they activate the channel from the vacuolar side. This is a crucial issue due to malate concentrations being in the EC 50 range in the cytosol but not in the vacuole [25] , [26] , [27] . To address this question, we used a pharmacological approach ( Fig. 2f ). We tested whether isophtalate, a malate analogue that does not permeate through AtALMT9 ( Supplementary Fig. S4 ) was able to activate chloride currents from the cytosolic side. Indeed, isophtalate was able to trigger the activation of AtALMT9 inducing a 2.1±0.1 fold increase of the chloride current at −120 mV ( Fig. 2f ). Moreover, cytosolic malate activates the AtALMT9 chloride currents even in presence of 100 mM malate in the vacuolar buffer ( Supplementary Fig. S5 ). These results strongly suggest that the interaction required to induce the activation of AtALMT9 occurs at the cytosolic side. 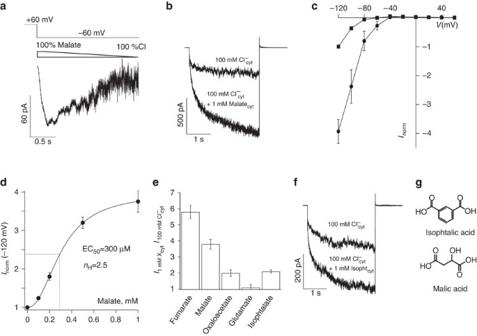Figure 2: Cytosolic malate activates AtALMT9-mediated chloride currents. (a) During the exchange of the cytosolic solution from 100 mM malatecytto 100 mM chloridecyt, the level of current fluctuation increases before the exchange is complete and the current amplitude reaches a steady state level. (b,c) In symmetrical chloride conditions (100 mM Clcyt−/100 mM Clvac−), the AtALMT9-mediated chloride currents increased by a factor of about 4 at −120 mV when 1 mM malate was added on the cytosolic side. Representative currents elicited in an excised cytosolic-side-out patch from an AtALMT9 overexpressing vacuole before (upper trace) and after the perfusion with 1 mM malate (lower trace) (b). NormalizedI–Vcurves of AtALMT9-mediated chloride currents in absence (squares;n=5) or in presence of 1 mM malatecyt(circles;n=5) (c;Supplementary Fig. S10, non-normalizedI–Vcurves). (d) Dose–response curve of the activation of AtALMT9-mediated chloride currents by cytosolic malate at −120 mV. Fitting the data with a Hill equation led to a Hill coefficient (nH) of 2.5 and an EC50of 300 μM (n=5–7). (e) Different dicarboxylic acids activate AtALMT9 with different potency while glutamate is not effective; all compounds were tested at a cytosolic concentration of 1 mM (n=5–9). (f) The interacting site responsible for the activation of AtALMT9 resides at the cytosolic side. Isophthalic acid, a dicarboxylic acid not permeable across AtALMT9 (Supplementary Fig. S4), is able to activate AtALMT9 currents. (g) Comparison of the molecular structures of Isophthalic acid and malic acid. (b,f) Currents evoked in response 3-s pulse at −120 mV followed by a tail pulse at +60 mV, holding potential +60 mV. Error bars are s.e.m. Figure 2: Cytosolic malate activates AtALMT9-mediated chloride currents. ( a ) During the exchange of the cytosolic solution from 100 mM malate cyt to 100 mM chloride cyt , the level of current fluctuation increases before the exchange is complete and the current amplitude reaches a steady state level. ( b , c ) In symmetrical chloride conditions (100 mM Cl cyt − /100 mM Cl vac − ), the AtALMT9-mediated chloride currents increased by a factor of about 4 at −120 mV when 1 mM malate was added on the cytosolic side. Representative currents elicited in an excised cytosolic-side-out patch from an AtALMT9 overexpressing vacuole before (upper trace) and after the perfusion with 1 mM malate (lower trace) ( b ). Normalized I – V curves of AtALMT9-mediated chloride currents in absence (squares; n =5) or in presence of 1 mM malate cyt (circles; n =5) ( c ; Supplementary Fig. S10 , non-normalized I – V curves). ( d ) Dose–response curve of the activation of AtALMT9-mediated chloride currents by cytosolic malate at −120 mV. Fitting the data with a Hill equation led to a Hill coefficient ( n H ) of 2.5 and an EC 50 of 300 μM ( n =5–7). ( e ) Different dicarboxylic acids activate AtALMT9 with different potency while glutamate is not effective; all compounds were tested at a cytosolic concentration of 1 mM ( n =5–9). ( f ) The interacting site responsible for the activation of AtALMT9 resides at the cytosolic side. Isophthalic acid, a dicarboxylic acid not permeable across AtALMT9 ( Supplementary Fig. S4 ), is able to activate AtALMT9 currents. ( g ) Comparison of the molecular structures of Isophthalic acid and malic acid. ( b , f ) Currents evoked in response 3-s pulse at −120 mV followed by a tail pulse at +60 mV, holding potential +60 mV. Error bars are s.e.m. Full size image Cytosolic malate increases AtALMT9 open probability The activation of chloride currents by carboxylates can be explained either by an increase of the single-channel conductance and/or the open probability. To answer this question, we performed a single-channel analysis of AtALMT9 ( Fig. 3 ). In excised out-side-out patches from vacuoles overexpressing AtALMT9-GFP, we could identify single-channel transitions with a conductance of 32±2 pS ( n =4) using conditions identical to those for macroscopic chloride current recordings ( Fig. 3a ). The single-channel amplitude was −3.9±0.2 pA at −120 mV ( Fig. 3b ), a value corresponding to that determined by non-stationary noise analysis of the macroscopic currents at the same voltage (−3.4±0.8 pA at −120 mV; Supplementary Fig. S6 ). The reversal potential of the single channels was 0±2 mV, which is very close to the Nernst potential for chloride ( E Nernst (Cl − )=0 mV). The open probability of the single-channel transitions was voltage dependent and increased at more negative voltages, which is in agreement with the macroscopic currents measurements ( Fig. 1a ). Under our experimental conditions, the single channels presented a flickery behaviour characterized by fast transitions between the open and the closed state ( Fig. 3a ), which explains the characteristic noisy behaviour of the macroscopic chloride currents ( Fig. 1 ). Notably, the characteristics of our single-channel measurements are comparable to the only available measurements of chloride single channels in the vacuolar membrane of higher plants reported so far [21] . This channel also, exhibited a flickery behaviour and a conductance of 34 pS (ref. 21 ). Next, we tested how the single-channel activity was altered by the addition of malate at the cytosolic side ( Fig. 3c ). We perfused patches in which single channels could be visualized with the chloride solution including 200 μM malate ( n =4; Fig. 3c ). All-point histograms revealed that 200 μM malate dramatically increased the open probability of AtALMT9 ( Fig. 3c ). Moreover, all-point histograms could be fitted by a sum of Gaussian functions that were equally spaced indicating that malate activation does not induce a change in the single-channel conductivity ( Fig. 3c ). This is supported by the observation that single-channel transitions detected in presence of malate displayed the same amplitude (−2.8±0.4 pA at −80 mV) as in the absence of cytosolic malate (−2.7±0.3 pA at −80 mV; Fig. 3c , inset). All together these data show that the single-channel activity observed can be attributed to AtALMT9. In addition, these results are also a final proof that ALMTs are channels and not transporters. 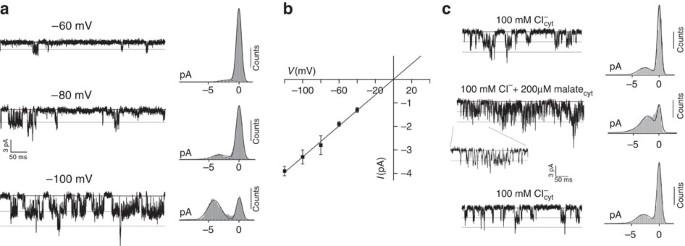Figure 3: Single-channel analysis of AtALMT9-mediated chloride currents. (a) Representative single-channel recordings at different applied membrane potentials as indicated. Single channels were measured in vacuolar patches from AtALMT9 overexpressing plants in symmetrical chloride conditions (100 mM Clcyt−/100 mM Clvac−). Corresponding all-point amplitude histograms of the single-channel recordings (right) show that the open probability increases when the applied membrane potential is more negative. (b) Single-channel I-V curve obtained from all-point amplitude histograms as in (a) shows that AtALMT9 presents a single-channel conductance of 32 pS (n=3–5). (c) Single channels observed in conditions as inaare reversibly activated by 200 μM malate added at the cytosolic side. The activation by cytosolic malate does not alter the single-channel conductance (−2.8±0.4 pA at −80 mV, inset), but increases the open probability as illustrated by the corresponding all-point amplitude histograms (right). In all-point amplitude histograms (a,c), the continuous line represents the fit with an adequate sum of Gaussian distributions. Data are filtered at 1.5 kHz. Error bars are s.e.m. Figure 3: Single-channel analysis of AtALMT9-mediated chloride currents. ( a ) Representative single-channel recordings at different applied membrane potentials as indicated. Single channels were measured in vacuolar patches from AtALMT9 overexpressing plants in symmetrical chloride conditions (100 mM Cl cyt − /100 mM Cl vac − ). Corresponding all-point amplitude histograms of the single-channel recordings (right) show that the open probability increases when the applied membrane potential is more negative. ( b ) Single-channel I-V curve obtained from all-point amplitude histograms as in ( a ) shows that AtALMT9 presents a single-channel conductance of 32 pS ( n =3–5). ( c ) Single channels observed in conditions as in a are reversibly activated by 200 μM malate added at the cytosolic side. The activation by cytosolic malate does not alter the single-channel conductance (−2.8±0.4 pA at −80 mV, inset), but increases the open probability as illustrated by the corresponding all-point amplitude histograms (right). In all-point amplitude histograms ( a , c ), the continuous line represents the fit with an adequate sum of Gaussian distributions. Data are filtered at 1.5 kHz. Error bars are s.e.m. Full size image AtALMT9 is a major vacuolar chloride channel We analysed whether the cytosolic malate activation of the chloride currents was observable also in A. thaliana vacuoles. Previously, it has been shown that vacuoles from mesophyll protoplasts display AtALMT9-mediated currents [18] , therefore we used this experimental system to test the malate activation in the native system. We designed experiments in which the buffer on the cytosolic side was sequentially exchanged in the following order: (i)100 mM Cl cyt − ; (ii) 100 mM Cl cyt − + 1 mM malate cyt ; (iii) 100 mM malate cyt , ( Fig. 4 ). In whole-vacuole recordings from Col-0, we could observe a reversible increase of 1.41±0.1 of the chloride currents after the addition of 1 mM malate ( Fig. 4a ) and an increase of the noise. The mean current densities at −120 mV in the different conditions were: −5.3±0.6 pA pF −1 in 100 mM Cl cyt − ; −7.4±0.9 pA pF −1 in 100 mM Cl cyt − +1 mM malate cyt ; −11.6±2.0 pA pF −1 in 100 mM malate cyt ; ( Fig. 4a ). We performed the same experiments using two AtALMT9 knockout lines, atalmt9-1 and atalmt9-2 ( Fig. 4 ). Neither in atalmt9-1 nor in atalmt9-2 an increase of the chloride currents was observed ( Fig. 4b ). The mean current densities at −120 mV in the knockout lines were: 100 mM Cl cyt − , atalmt9-1 −4.4±0.4 pA pF −1 , atalmt9-2 −3.8±0.5 pA pF −1 ; 100 mM Cl cyt − +1 mM malate cyt , atalmt9-1 −4.5±0.5 pA pF −1 , atalmt9-2 −3.7±0.5 pA pF −1 ; 100 mM malate cyt , atalmt9-1 −2.1±0.4 pA pF −1 , atalmt9-1 −2.8±0.4 pA pF −1 ; ( Fig. 4b ). The absence of the cytosolic malate activation of the chloride currents in both the knockouts demonstrates that the increase induced by cytosolic malate we observed in Col-0 is due to AtALMT9. Moreover, the absence of the malate activation in atalmt9-1 and atalmt9-2 is followed by a dramatic decrease of the current density observed in presence of 100 mM malate in the cytosol. 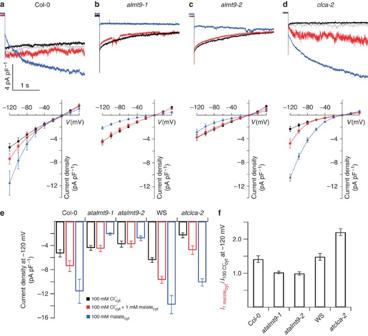Figure 4: Cytosolic malate activates chloride currents inA. thalianavacuoles from mesophyll protoplasts. Representative current recordings (upper panel; at −120 mV) and meanI–Vcurves normalized to the capacitance (lower panel) obtained in whole-vacuole configuration: (a) Col-0 out-crossed wild-type (n=10), (b)atalmt9-1(n=5), (c)atalmt9-2(n=6) and (d)atclca-2(n=6) knockout lines during cytosolic solution exchange. Black, 100 mM Clcyt−/100 mM Clvac−; red, 100 mM Clcyt−+1 mM malatecyt/100 mM Clvac−; blue, 100 mM malatecyt/100 mM malatevac; grey, recovery. In the wild-type vacuoles (a), the addition of 1 mM malatecytinduces a reversible increase of the chloride currents of 1.43 times atVm=−120 mV while in theatalmt9-1(b) and2(c) no activation of the chloride currents is observable. (d) theatclca-2knockout mutant presents a decreased anionic current background and an increase of the chloride currents in response to 1 mM malatecytof 2.2 times at −120 mV. (e) Mean current density atVm=−120 mV of the different genotypes in the different tested conditions. (f) Ratio of the current measured in 100 mM Clcyt−+ 1 mM malatecytand the current measured in 100 mM Clcyt−for the different genotypes. Ineandf, results from wild-type Wassilewskija (WS;n=4) are shown. (a–d) Currents evoked in response 3-s pulse from +60 mV to −120 mV, holding potential +60 mV.I–Vcharacteristics were obtained averaging the last 50 ms of the current traces. Error bars are s.e.m. Figure 4: Cytosolic malate activates chloride currents in A. thaliana vacuoles from mesophyll protoplasts. Representative current recordings (upper panel; at −120 mV) and mean I – V curves normalized to the capacitance (lower panel) obtained in whole-vacuole configuration: ( a ) Col-0 out-crossed wild-type ( n =10), ( b ) atalmt9-1 ( n =5), ( c ) atalmt9-2 ( n =6) and ( d ) atclca-2 ( n =6) knockout lines during cytosolic solution exchange. Black, 100 mM Cl cyt − /100 mM Cl vac − ; red, 100 mM Cl cyt − +1 mM malate cyt /100 mM Cl vac − ; blue, 100 mM malate cyt /100 mM malate vac ; grey, recovery. In the wild-type vacuoles ( a ), the addition of 1 mM malate cyt induces a reversible increase of the chloride currents of 1.43 times at V m =−120 mV while in the atalmt9-1 ( b ) and 2 ( c ) no activation of the chloride currents is observable. ( d ) the atclca-2 knockout mutant presents a decreased anionic current background and an increase of the chloride currents in response to 1 mM malate cyt of 2.2 times at −120 mV. ( e ) Mean current density at V m =−120 mV of the different genotypes in the different tested conditions. ( f ) Ratio of the current measured in 100 mM Cl cyt − + 1 mM malate cyt and the current measured in 100 mM Cl cyt − for the different genotypes. In e and f , results from wild-type Wassilewskija (WS; n =4) are shown. ( a – d ) Currents evoked in response 3-s pulse from +60 mV to −120 mV, holding potential +60 mV. I – V characteristics were obtained averaging the last 50 ms of the current traces. Error bars are s.e.m. Full size image Despite the fact that we could measure consistent malate activation in wild-type vacuoles, we were puzzled by the smaller extent of the activation compared with that observed in AtALMT9 overexpressing N. benthamiana vacuoles. We hypothesized that in our Arabidopsis , whole-vacuole measurements there was a background chloride current independent from other vacuolar ALMTs masking the malate activation, which would consequently result in a reduced effect of cytosolic malate. AtCLCa has been shown to mediate the main inorganic anion current across the Arabidopsis tonoplast and to be able to transport NO 3 − (ref. 12 ) but also Cl − (ref. 29 ). We found that in the presence of 100 mM Cl cyt − vacuoles from atclca-2 exhibited a current density of −2.3±0.4 pA pF −1 ( Fig. 4d ) compared with the −6.4±0.4 pA pF −1 observed in the corresponding wild type (WS, Wassilewskija). This result shows that atclca-2 actually present a strongly diminished background chloride current compared with the wild type ( Fig. 4e ). When the 100 mM Cl cyt − +1 mM malate cyt buffer was applied in atclca-2 , the current increased by a similar amount as in the wild type. However, as the contribution of AtCLCa was no more present, the activation by malate was increased by a factor of 2.2±0.1 compared with 1.48±0.1 in WS, showing that the reduced background of atclca-2 resulted in an increased activation effect of malate cyt . These results show that the reduced activation of the chloride currents by 1 mM cytosolic malate in wild-type Arabidopsis vacuoles ( Fig. 4a ) compared with the activation measured in overexpressing tobacco vacuoles is likely to be due to the higher relative contribution of background chloride currents in Arabidopsis . AtALMT9 controls stomata aperture As chloride ions are known to have a major role in stomatal movements in Arabidopsis , we investigated whether and how AtALMT9 could be involved in this process. Coinciding with in silico data (Genevestigator, http://www.genevestigator.ethz.ch ), experiments using plants expressing GUS under the control of the AtALMT9 promoter confirmed that this channel is also expressed in guard cells ( Fig. 5a ). As the currents mediated by AtALMT9 were strongly inward rectifying, we expected a physiological role of AtALMT9 in the opening process of stomata. Indeed, the closure induced by dark or ABA is not impaired in atalmt9 mutants ( Supplementary Fig. S7 ). Therefore we performed stomatal opening assays on peeled epidermal strips from two independent atalmt9 knockout lines using a 30 mM KCl buffer ( Fig. 5b ). After exposure to light for 2 h, we could detect a 20% and 21%, reduced stomatal aperture in the atalmt9-1 and atalmt9-2 mutants, respectively ( Fig. 5c ). Interestingly, when the same assay was made in presence of 3 mM Cl − (30 mM K + , 3 mM Cl − and 27 mM iminodiacetate), the stomata aperture after the exposure to 2 h light of both wild types and mutants was similar but reduced compared to that of wild type in 30 mM KCl ( Fig. 5c ). Guard cells accumulate different anions such as malate and Cl − during stomata opening to balance K + charges [4] , [5] , [6] . The relative accumulation of Cl − and malate in the vacuole depends on the availability of chloride [10] , [30] . In this context, our data indicate that AtALMT9 is involved in mediating chloride fluxes in the vacuole of guard cells to achieve a complete stomata opening. 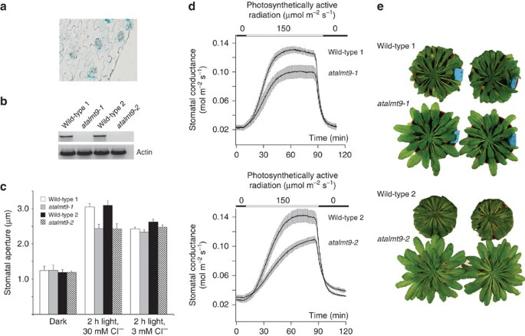Figure 5: AtALMT9 is involved in stomatal opening inA. thaliana. (a)AtALMT9-promoter-GUS reporter lines show that AtALMT9 is expressed in guard cells. (b) Two independent knockout mutant lines,atalmt9-1andatalmt9-2(for details see material and methods), were used to determine the role of the AtALMT9 chloride channel in stomatal opening. In both lines, RNA transcripts for AtALMT9 could not be detected. (c) Stomatal aperture measurements on stripped epidermis after 2 h of illuminationatalmt9-1andatalmt9-2knockout mutants and wild-type plants. Measurements performed in presence of 30 mM KCl show that the knockout mutants presented a decreased aperture of 20±3% (atalmt9-1,P=0.004t-test;n=6) and 21±4% (atalmt9-2, P=0.003t-test;n=6) with respect to the corresponding wild types. Measurements performed in presence of 27 mM K-Iminodiacetate and 3 mM KCl show thatatalmt9-1andatalmt9-2knockout mutants do not show significant difference in stomatal apertures (atalmt9-1, P=0.11t-test;atalmt9-2, P=0.21t-test). Each point corresponds to the mean of six experiments, in each experiment at least 60 stomata were analysed. (d) Time course of the mean stomatal conductance during light-induced opening. Measurements were performed using a LI-6400; LI-COR gas exchange chamber. It is visible that in bothatalmt9-1(upper panel;atalmt9-1,n=6 plants; wild-type-1,n=5 plants) andatalmt9-2(lower panel;atalmt9-2,n=6 plants; wild-type-2,n=6 plants) knockouts, the stomatal conductance increase is delayed compared with the corresponding wild-type plants. After 1.5 h, the two knockout lines reach a lower conductance level (atalmt9-122%;atalmt9-225%) than the corresponding wild types. (e)atalmt9-1andatalmt9-2are more tolerant to drought, 8 days after stopping wateringatalmt9-1(upper panel) andatalmt9-2(lower panel) are still turgescent, while the corresponding wild types are withered. Error bars are s.e.m. Figure 5: AtALMT9 is involved in stomatal opening in A. thaliana . ( a ) AtALMT9 -promoter-GUS reporter lines show that AtALMT9 is expressed in guard cells. ( b ) Two independent knockout mutant lines, atalmt9-1 and atalmt9-2 (for details see material and methods), were used to determine the role of the AtALMT9 chloride channel in stomatal opening. In both lines, RNA transcripts for AtALMT9 could not be detected. ( c ) Stomatal aperture measurements on stripped epidermis after 2 h of illumination atalmt9-1 and atalmt9-2 knockout mutants and wild-type plants. Measurements performed in presence of 30 mM KCl show that the knockout mutants presented a decreased aperture of 20±3% ( atalmt9-1 , P =0.004 t -test; n =6) and 21±4% ( atalmt9-2, P =0.003 t -test; n =6) with respect to the corresponding wild types. Measurements performed in presence of 27 mM K-Iminodiacetate and 3 mM KCl show that atalmt9-1 and atalmt9-2 knockout mutants do not show significant difference in stomatal apertures ( atalmt9-1, P =0.11 t -test; atalmt9-2, P =0.21 t -test). Each point corresponds to the mean of six experiments, in each experiment at least 60 stomata were analysed. ( d ) Time course of the mean stomatal conductance during light-induced opening. Measurements were performed using a LI-6400; LI-COR gas exchange chamber. It is visible that in both atalmt9-1 (upper panel; atalmt9-1 , n =6 plants; wild-type-1, n =5 plants) and atalmt9-2 (lower panel; atalmt9-2 , n =6 plants; wild-type-2, n =6 plants) knockouts, the stomatal conductance increase is delayed compared with the corresponding wild-type plants. After 1.5 h, the two knockout lines reach a lower conductance level ( atalmt9-1 22%; atalmt9-2 25%) than the corresponding wild types. ( e ) atalmt9-1 and atalmt9-2 are more tolerant to drought, 8 days after stopping watering atalmt9-1 (upper panel) and atalmt9-2 (lower panel) are still turgescent, while the corresponding wild types are withered. Error bars are s.e.m. Full size image Furthermore, we monitored the kinetics of stomatal opening in Arabidopsis leaves by measuring changes in the stomatal conductance in response to light ( Fig. 5d , Supplementary Fig. S8 ). Compared with wild-type plants, stomatal conductance was lower after 100 min of light exposure in both atalmt9 knockout lines and measurements revealed significantly slower opening kinetics in the mutants than in the wild-type plants. To obtain further evidences that loss of AtALMT9 affects also stomatal opening in planta , we exposed wild type and knockout plants to drought stress ( Fig. 5e ). Both knockout lines were more resistant to drought compared with the corresponding wild-type lines. At 8 days after the last watering, wild-type plants had 23% lower water content compared with the corresponding knockout lines ( Supplementary Fig. S9 ). Like in previous studies, no visual phenotype on leaves was observed [18] . However, to verify that the drought stress phenotype was not due to a rapid hydropassive water loss, we measured the osmolarity of wild type and knockout mutants. As expected from the similar water content in both lines, the osmolarity of the press sap was also indistinguishable. These results indicate that the increased drought resistance of atalmt9- 1 and atalmt9-2 is not due to a less negative water potential in the mutant ( Supplementary Fig. S9 ) but to the impaired stomatal opening ( Fig. 5c ). To guarantee appropriate gas exchanges under changing environmental conditions, ion transport and metabolism have to be integrated processes in guard cells. Anions have to meet the metabolic requirements of the cell as well as to keep the ionic balance and the osmotic potential. Chloride has an important role as an osmoticum and charge balance but is metabolically inactive. In contrast, malate is part of several metabolic pathways and through the action on PEPcase regulates the synthesis of oxaloacetate, its precursor [31] . During stomatal opening concomitantly to potassium uptake, malate and chloride are taken up from the apoplast [1] , [4] , [6] , [32] . Moreover, malate is also synthesized via starch degradation [4] , [5] . The amount of malate in the apoplast is limited and the synthesis of large amounts of malate through starch breakdown and glycolysis is likely to be slower than the uptake. As the cytosolic volume of guard cells is only about 20–30% of the cellular volume when stomata are closed, small increases of cytosolic malate are sufficient to activate the vacuolar chloride channel and consequently allow a rapid opening reaction via chloride accumulation in the vacuole. Consequently, at least in short terms, malate may not have the role as the main osmolyte during stomatal opening but rather exhibit a so far unexplored signalling function: the regulation of anion fluxes across the plasma and the vacuolar membranes, hence participating in the control of the osmotic pressure of guard cells ( Fig. 6 ). We found that AtALMT9 mediates chloride currents activated by cytosolic malate in a physiological concentration range in both heterologous expression system and under native conditions. In Arabidopsis , the relative contribution of AtALMT9 in vacuolar chloride fluxes can be estimated based on our data. We could attribute the relatively weak activation observed in Arabidopsis compared with the measurements in N. benthamiana overexpressing AtALMT9 to the relative high background currents in Arabidopsis vacuoles. However, taking the measured values and deducing the background current by calculating the ratios of (( I Cl+mal Col−0 − I Cl+mal almt9 )/( I Cl Col−0 − I Cl almt9 )), an activation of the AtALMT9-mediated chloride current of ~3 could be obtained; a value similar to that observed in tobacco. 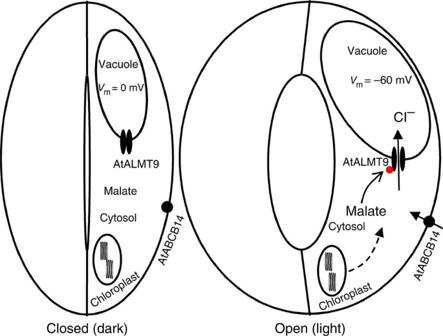Figure 6: Model for the role of AtALMT9 in stomatal opening. When stomata are closed (at the end of the dark period), the vacuolar membrane potential is close to 0 mV and cytosolic malate concentrations are low (left panel). In these conditions, AtALMT9 is not active and does mediate anion accumulation into the vacuole. During stomatal opening (right panel), the membrane potential of the vacuole drops to values close to −60 mV. Starch is degraded to malate, which is also taken up from the apoplast inducing a raise of the cytosolic malate concentration. These conditions activate AtALMT9. At the same time, chloride enters into guard cells. To sustain the opening of stomata, solutes have to be accumulated in the vacuole of guard cells to increase the water potential. In this phase, AtALMT9 mediates chloride accumulation in the vacuole. Figure 6: Model for the role of AtALMT9 in stomatal opening. When stomata are closed (at the end of the dark period), the vacuolar membrane potential is close to 0 mV and cytosolic malate concentrations are low (left panel). In these conditions, AtALMT9 is not active and does mediate anion accumulation into the vacuole. During stomatal opening (right panel), the membrane potential of the vacuole drops to values close to −60 mV. Starch is degraded to malate, which is also taken up from the apoplast inducing a raise of the cytosolic malate concentration. These conditions activate AtALMT9. At the same time, chloride enters into guard cells. To sustain the opening of stomata, solutes have to be accumulated in the vacuole of guard cells to increase the water potential. In this phase, AtALMT9 mediates chloride accumulation in the vacuole. Full size image At −120 mV and in the presence of 100 mM Cl − , and 1 mM malate the current through AtALMT9 is ~−3 pA pF −1 . We found that beside AtALMT9 the major current under our experimental conditions is generated by AtCLCa with a current density of ~−3 pA pFA −1 . If one takes into account that AtCLCa is a nitrate, chloride/proton antiporter [12] , [29] and that under our experimental conditions, two protons are exported for each chloride taken up by the vacuole it results that the chloride flux mediated by AtALMT9 is about three times the one mediated by AtCLCa. Nonetheless, it should be mentioned that the relative contributions of AtALMT9 and AtCLCa may differ in function of the given membrane potential and cytosolic chloride concentrations and regulatory factors. Our results also show that AtALMT9 is required for fast and complete opening of stomata, but has no effect on stomata closure. Mutants of AtALMT9 wilt faster, which is in accordance with the gas exchange data and the measurements made on isolated epidermal strips. AtALMT9 is also expressed in the mesophyll cells [18] . To exclude indirect effect of the mesophyll, we compared water contents and the osmolarity in the leaves of wild-type and mutant plants. Both parameters were displaying no significant differences between wild-type and knockout plants consequently excluding a role of the mesophyll in the observed phenotype. Therefore, the drought-resistant phenotype of the knockout can be attributed to the impaired stomatal opening resulting from a reduced uptake of chloride in guard cell vacuoles. This is in line with the functional properties of AtALMT9 mediating chloride fluxes directed into the vacuole. Wang and Blatt [33] have recently shown that carboxylates inhibit chloride fluxes across the plasma membrane of Vicia faba guard cells, indicating that carboxylates act as important regulatory elements of chloride fluxes across cellular membranes. In our work, we identified AtALMT9 as target of the carboxylate modulation. Whether the inhibition observed by Wang and Blatt [33] is due to an opposite regulatory effect of carboxylates on plasma membrane localized ALMTs or SLACs or whether an inhibition of the plasma membrane chloride efflux was observed due to the activation of the vacuolar chloride currents remains to be established. The discovery that AtALMT9 constitutes a vacuolar chloride channel, which has been sought for over 20 years, assigns a completely novel function to this anion channel. These results may pave the way to get further insights in the regulation of guard cell anion channels and finally to modulate stomatal aperture allowing to produce plants that are more drought tolerant and more productive under certain environmental conditions. Overexpression of AtALMT9-GFP in Nicotiana benthamiana For transient overexpression of AtALMT9-GFP, the complementary DNA was cloned into the pART27 vector as described previously [18] .The agrobacterium-mediated infiltration of N. benthamiana leaves was perfomed as described [34] with slight modifications. After agrobacterium-mediated infiltration tobacco plants were grown in greenhouse (16 h light:8 h dark, 25 °C). At 2–3 days after the agrobacterium-mediated infiltration, the transformed leaves were used to extract protoplasts and vacuoles for patch-clamp experiments. Electrophysiology Mesophyll protoplasts from tobacco leaves were released by an enzymatic digestion. The enzyme solution contained 0.3% (w/v) cellulase R-10, 0.03% (w/v) pectolyase Y-23, 1 mM CaCl 2 , 500 mM sorbitol and 10 mM MES, pH 5.3 (550 mOsm). Protoplasts were washed twice and resuspended in the same solution without enzymes. Vacuoles were released from mesophyll protoplast by the addition of 5 mM EDTA and a slight osmotic shock (500 mOsm, see medium below). Vacuoles from transformed protoplasts to be used for patch-clamp experiments were selected using an epifluorescence microscope. Membrane currents from tonoplast patches were recorded using the patch-clamp technique [12] , [19] . Briefly, currents were recorded with an EPC10 patch-clamp amplifier (HEKA Electronics) using the Patchmaster software (HEKA Electronics). Data were analysed with the FitMaster software (HEKA Electronics). Exchange of the cytosolic-side solution was performed using a gravity-driven perfusion system. In experiments on macroscopic currents recording and whole-vacuole, the pipette resistance was 4–5 MΩ. For single-channel recordings, the pipette resistance was 8–9 MΩ. Only patches presenting a seal resistance higher than 2 GΩ for macroscopic currents and 8–10 GΩ for single-channel recordings were used to perform experiments. In whole-vacuole recordings, to equilibrate the vacuolar lumen with the pipette solution, at least 10 min were waited after the establishment of the whole-vacuole configuration before starting the exchange of the cytosolic-side solution. Current recordings were filtered at 300 Hz for macroscopic currents and 1.5 kHz for single-channel recordings. The pipette solutions contained: 112 mM malic acid, 5 mM HCl, adjusted with BisTrisPropane, pH 6; 100 mM HCl, adjusted to pH 6 with BisTrisPropane. The osmolarity was adjusted to 550 mOsm with sorbitol. The bath solutions contained: (i) 100 mM malic acid, 3 mM MgCl 2 , 0.1 mM CaCl 2 , adjusted to pH 7.5 with BisTrisPropane; (ii) 100 mM HCl, 3 mM MgCl 2 , 0.1 mM CaCl 2 , adjusted to pH 7.5 with BisTrisPropane. The osmolarity was adjusted to 500 mOsm with sorbitol. For activation experiments of the chloride currents, the dicarboxylic acids (malic acid, isophthalic acid, fumaric acid, oxaloacetic acid and glutamic acid) were added to the chloride-based bath solution at the concentrations indicated in the text. When needed the pH was adjusted to 7.5 with BisTrisPropane. All chemicals were purchased at Sigma-Aldrich. Liquid junction potentials were measured [35] and corrected when higher that ±2 mV. When not stated differently the current–voltage characteristics were obtained by subtracting the current at t =0 from the quasi-stationary currents (averaging the last 50 ms of the current trace) elicited by main voltage pulses. For the channel activation by malate, the concentration-dependent activation relationship was fitted by the Hill equation in the form of: where I act is the current in presence of the activator, I ctrl is the current in absence of the activator. n H is the Hill coefficient and [act] is the concentration of the activator. K A is the EC50. A is the maximum current ratio. Plant material and growth conditions. All wild type (Col-0) and atalmt9 mutant plants of Arabidopsis thaliana were grown in a plant growth chamber (8 h light 22 °C/16 h dark 18 °C, 55% relative humidity) in potting soil. For drought stress experiments, plants were grown in a defined amount of sieved soil in round pots (6 cm diameter). After 8 weeks of regular irrigation, watering was stopped. Selection of atalmt9 knockout lines Two independent T-DNA insertion lines, atalmt9-1 (SALK_055490) and atalmt9-2 (WiscDsLox499H09), were obtained from the Salk Institute Genomic Analysis Laboratory and the Wisconsin Arabidopsis T-DNA insertion collection, respectively. Genomic DNA was extracted from 4-week-old plants and mutant plants homozygous for the T-DNA insertion locus were isolated by PCR genotyping using AtALMT9 -specific primers. To select homozygous lines, we used the AtALMT9 -specific primer At3g18440-solfor (5′-GATCCTGCAGGCTGGAGAGGATCTTCATAACCTTG-3′) and At3g18440–solrev (5′-GATCGCGGCCGCTTACATCCCAAAACACCTACGAATC-3′) and the T-DNA-specific primer LBb1.3 (5′-ATTTTGCCGATTTCGGAAC-3′) and p745 (5′-AACGTCCGCAATGTGTTATTAAGTTGTC-3′) for atalmt9-1 and 2 , respectively. The abundance of the AtALMT9 transcript in homozygous knockout lines and wild-type plants (see below) was assayed by reverse transcriptase–PCR using the AtALMT9 -specific primers ALMT9-1F (5′-CCTTAATTAAATGGCGGCGAAGCAAGGTTCCTTCA-3′) and ALMT9-1794R (5′-TTGGCGCGCCCATCCCAAAACAC CTACGAATCT-3′). As loading control, actin transcript was amplified with the primers 5′-TGGAATCCACGAGACAACCT-3′ and 5′-TTCTGTGAACGATTCCTGGAC-3′. Stomatal aperture and gas exchange measurements Stomatal aperture and conductance were assayed from leaves of 5- to 7-week-old plants. Stomatal conductances of wild-type, atalmt9-1 and atalmt9-2 plants were measured using a portable gas exchange system (LI-6400; LI-COR) with an Arabidopsis leaf chamber fluorometer (LI-6400-40, LI-COR) and a light source set to 150 μmol m −2 s −1 (10% blue light). The relative humidity of incoming air was 58%±2% and the air flow was set to 300 μmol s −1 . For stomatal aperture measurement, the whole leaf was detached in the dark before start of the light period and glued from the abaxial side onto a coverslip using a non-toxic medical adhesive (Medical Adhesive B Liquid, VM 355-1, Ulrich Swiss). The adaxial epidermis and mesophyll layers were gently removed. The coverslips with the glued abaxial epidermis were placed in a Petri dish containing the opening buffer. The 30 mM Cl − buffer contains: 30 mM KCl, 5 mM MES, 0.1 mM CaCl 2 , pH 5.7. The 3 mM Cl − buffer contains: 3 mM KCl, 13.5 mM K 2 Iminodiacetate,0.1 mM CaCl 2 , pH 5.7. The epidermis was equilibrated for 30 min in dark ( t =0) and then incubated for 2 h in light. Wild-type and knockout leaves were analysed in parallel. Around 20 pictures per leaf and per time point were taken using an inverted microscope (Nikon Eclipse TS100) at a × 40 magnification. Stomatal apertures were measured manually using the ImageJ software. For each time point, more than 60 stomatal apertures were measured. Tissue-specific expression of AtALMT9 in Arabidopsis For GUS staining, the whole leaf was detached from the same transgenic plants lines as described (1). The abaxial epidermis was peeled and incubated in GUS staining buffer (50 mM NaHPO 4 pH 7.2, 0.5% Triton X-100, 1 mM X-Gluc) at 37 °C for 30 h, subsequently the GUS staining buffer was replaced with 70% ethanol. The samples were examined using a Nikon Eclipse TS100 microscope. How to cite this article: De Angeli, A. et al . AtALMT9 is a malate-activated vacuolar chloride channel required for stomatal opening in Arabidopsis . Nat. Commun. 3:1804 doi: 10.1038/ncomms2815 (2013).